Emulating weak localization using a solid-state quantum circuit Quantum interference is one of the most fundamental physical effects found in nature. Recent advances in quantum computing now employ interference as a fundamental resource for computation and control. Quantum interference also lies at the heart of sophisticated condensed matter phenomena such as Anderson localization, phenomena that are difficult to reproduce in numerical simulations. Here, employing a multiple-element superconducting quantum circuit, with which we manipulate a single microwave photon, we demonstrate that we can emulate the basic effects of weak localization. By engineering the control sequence, we are able to reproduce the well-known negative magnetoresistance of weak localization as well as its temperature dependence. Furthermore, we can use our circuit to continuously tune the level of disorder, a parameter that is not readily accessible in mesoscopic systems. Demonstrating a high level of control, our experiment shows the potential for employing superconducting quantum circuits as emulators for complex quantum phenomena. Superconducting qubits now demonstrate coherence times roughly one thousand times the single- and two-qubit gate times [1] , achieved using planar lithographically patterned circuits that can easily be scaled up to large numbers of qubits. As a result, this platform holds great promise for building a large-scale quantum computer [2] , [3] . These advantages also apply to the construction of quantum simulators [4] , [5] , [6] , [7] , [8] , [9] , [10] , [11] , for which demonstrations have been made on different problems [12] , [13] , [14] . Here, we use a multi-qubit circuit to demonstrate quantum emulation of weak localization, one of the most surprising manifestations of quantum interference in disordered mesoscopic systems. Weak localization results from the enhanced backscattering of electrons travelling in a weakly disordered medium [15] . Given the reasonably long coherence distances for electrons in such media, an electron can simultaneously follow multiple trajectories that can interfere constructively or destructively, depending on the details of the scattering path as well as external parameters such as magnetic field. The probability for the electron to reach a certain point is given by where the first term sums over classical probabilities and the second represents quantum interference. The random scattering events an electron undergoes randomize its wavevector, so that the second term typically averages to zero, leaving the classically determined probability for an electron to reach a certain point. A dominant exception to this is due to closed trajectories, where the electron returns to its starting point, as in the absence of energy loss, these trajectories always have a time-reversed counterpart with identical accumulated phase. As a result, direct and time-reversed paths interfere constructively with one another, yielding a probability for a closed path that is twice the classically expected value, increasing the electrical resistance (see Fig. 1a ). This constructive interference can, however, be reduced by applying an external magnetic field, so the measured electrical resistance is a maximum at zero applied field and falls to the classical resistance value as the magnetic field is increased—a hallmark of weak localization. Weak localization also has a very characteristic temperature dependence, as elevating the temperature increases the inelastic scattering rate, thereby suppressing the constructive interference and reducing the weak localization resistance peak [15] , [16] . 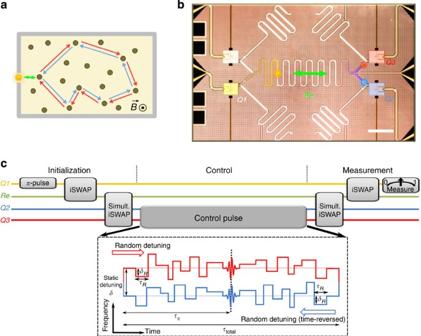Figure 1: Emulation of weak localization using superconducting quantum circuit. (a) Schematic illustrating the basic physics of weak localization. The weak localization contribution to the electrical resistance is dominated by the interference between closed trajectories traversed in opposite directions, which in the small decoherence limit give an increase in the resistance; here we show one such pair of trajectories. (b) Micrograph of the superconducting quantum circuit used to emulate weak localization. A single microwave excitation is generated in qubitQ1, distributed betweenQ2 andQ3 and the coupling resonatorRe, then manipulated in the simulation. Scale bar, 500 μm (c) Pulse sequence used to emulate weak localization, decomposed into three steps: Initialization: Aπ-pulse creates an excitation inQ1 that is then swapped into resonatorRethrough aniSWAP gate. A second simultaneousiSWAP gate then transfers the excitation fromReequally toQ2 andQ3 through their three-body interaction, creating the entangled state. Control: We apply toQ2 a relative static detuningδ, as well as a sequence of random detuningsδReach lasting for a random timeτR, interspersed with a refocusingπ-pulse delayed in time byτπto vary the effective coherence time. We apply the time-reversed sequence toQ3. Measurement: A simultaneousiSWAP interferes the states ofQ2 andQ3 inRe, and a secondiSWAP returns the excitation toQ1; the probability forQ1 to be in the excited state |e› is then measured. Figure 1: Emulation of weak localization using superconducting quantum circuit. ( a ) Schematic illustrating the basic physics of weak localization. The weak localization contribution to the electrical resistance is dominated by the interference between closed trajectories traversed in opposite directions, which in the small decoherence limit give an increase in the resistance; here we show one such pair of trajectories. ( b ) Micrograph of the superconducting quantum circuit used to emulate weak localization. A single microwave excitation is generated in qubit Q 1, distributed between Q 2 and Q 3 and the coupling resonator Re , then manipulated in the simulation. Scale bar, 500 μm ( c ) Pulse sequence used to emulate weak localization, decomposed into three steps: Initialization: A π -pulse creates an excitation in Q 1 that is then swapped into resonator Re through an i SWAP gate. A second simultaneous i SWAP gate then transfers the excitation from Re equally to Q 2 and Q 3 through their three-body interaction, creating the entangled state . Control: We apply to Q 2 a relative static detuning δ , as well as a sequence of random detunings δ R each lasting for a random time τ R , interspersed with a refocusing π -pulse delayed in time by τ π to vary the effective coherence time . We apply the time-reversed sequence to Q 3. Measurement: A simultaneous i SWAP interferes the states of Q 2 and Q 3 in Re , and a second i SWAP returns the excitation to Q 1; the probability for Q 1 to be in the excited state | e › is then measured. Full size image Given that quantum interference lies at the heart of weak localization, it is natural to use wave-like systems to emulate this effect. Demonstrations have been made in optical systems, where both coherent backscattering and transition to Anderson localization have been observed for optical photons travelling in disorder media [17] , [18] , [19] , [20] , [21] , [22] . In contrast to the optical counterpart, individual microwave photons in superconducting quantum circuits can be manipulated with a high degree of precision. Arbitrary control over the scattering processes allows for the investigation of more profound aspects of weak localization. Direct emulation is still a significant challenge, as the electrical resistance arises from the interference of many scattering trajectories [15] , thus requiring a very large superconducting emulator. The only notable demonstration to date was carried out with a single flux qubit, where a universal conductance fluctuation peak was emulated by asymmetrically driving the qubit through an avoided level crossing [23] . In the experiment reported here, we find that we can implement a controllable emulation of weak localization, using a small physical quantum simulator in a time-domain ensemble approach. We sequentially run through many different parameter sets for our quantum system, with each set representing a different pair of scattering trajectories in the mesoscopic system. Using an intuitive correspondence between the quantum circuit parameters and the mesoscopic system, we are able to map the spatial complexity of the mesoscopic system onto a set of complex yet manageable quantum control sequences in the time domain. In this way, we are able to illustrate the basics of the weak localization, using a few-element quantum circuit. Mapping electronic systems onto quantum circuits The quantum circuit used in this experiment comprises three phase qubits, a readout qubit Q1 and two control qubits Q2 and Q3 , symmetrically coupled to a bus resonator Re , as shown in Fig. 1b (ref. 24 ). In this configuration, the quantum circuit can be described by the Tavis–Cummings model [25] where ω i are the frequencies of the qubits i =1 to 3, ω r the resonator and g is the qubit–resonator coupling strength. The emulation was implemented by distributing the microwave photon into physically distinct circuit elements. In contrast with previous demonstrations using only a single qubit, multiple quantum elements allow us to separate backscattering from forward scattering. Despite small deviations in the qubit properties such as coherence, this technique may be readily applied to more complex quantum circuits, and thus provides a scalable method to emulate the effects of weak localization. As shown in Fig. 1c , we start the experiment by generating and then splitting a microwave photon in a superposition state between the two control qubits, analogous to an incoming electron simultaneously traversing two trajectories (see Supplementary Fig. 1 ). This was done by first initializing Q 1 in | e › with a microwave pulse and swapping the excitation into Re . By bringing Q 2 and Q 3 simultaneously on resonance with Re for a time , we execute a simultaneous i SWAP gate [24] , [26] that transfers the excitation from Re equally to the two control qubits through their three-body interaction, resulting in the desired state . Compared with the product state , the entangled state confines the emulation process within the single-excitation subspace, and therefore maximizes the signal-to-noise ratio of the experimental results. To emulate the diffusion process of an electron in a random medium, including the presence of a magnetic field, we use the mapping between mesoscopic transport and quantum circuit parameters delineated in Table 1 . The motion of the electron is emulated using a time-domain control sequence applied to each of the control qubits. To mimic the random scattering, we use a series of random frequency detunings , each lasting for a random duration (see the extended pulse sequence in Fig. 1c ). This results in a dynamic phase , resembling the random scattering phase of an electron with wavevector following a trajectory . Qubit Q 2 undergoes one set of random detunings, simulating a trajectory, while Q 3 is driven by the time-reversed sequence applied to Q 2, thereby simulating the time-reversed electron trajectory. In addition, we apply a static detuning δ throughout the entire process, resulting in a static phase φ S = δ · τ total between the two qubits. This resembles the magnetic field-induced phase shift , with δ and τ total corresponding to and , respectively. Table 1 Mapping between parameters for electrons in mesoscopic systems to control parameters of quantum circuits. Full size table To emulate the temperature dependence of weak localization, where changing the temperatures modifies the electron transport coherence length, we use the Table 1 mapping between the the electron phase coherence length L ϕ and the qubit effective coherence time ; we vary the effective coherence time by inserting a refocusing π -pulse into the qubit control sequence described above. Instead of the conventional Hahn-echo sequence [27] , with the refocusing pulse placed at τ π / τ total =1/2, we vary the timing of the refocusing pulse, such that the effective phase coherence time can be continuously varied from ~100 ns to >200 ns (measured by Ramsey-type experiments—see Supplementary Fig. 2 ). Following the application of this control sequence, we then interfere the microwave photon with itself and measure the outcome. To do this, we apply a second simultaneous i SWAP gate, which recombines and interferes the excitations in Q 2 and Q 3 in Re . Following this, an i SWAP brings the interference result from Re back to Q 1, with the probability of finding Q 1 in | e › corresponding to the return probability of the electron in the direct and reversed trajectories. To obtain statistically significant results, we sequentially run through 100 different control sequences, with different static and random detuning configurations, and average the qubit measurement outcomes to arrive at the average return probability P return , which in the emulation corresponds to the electrical resistance in mesoscopic transport. Emulating fundamentals of weak localization In Fig. 2a , we show the experimental P return versus static detuning δ for six different , corresponding to magnetoresistance measurements at six different temperatures. For all data sets, the probability P return has its maximum at δ =0, where time-reversal symmetry is protected. As δ moves away from zero, P return rapidly decreases until it reaches an average value of ~0.35, about which it fluctuates randomly. The reduction in P return with increasing | δ | is consistent with the well-known negative magnetoresistance in the mesoscopic system. 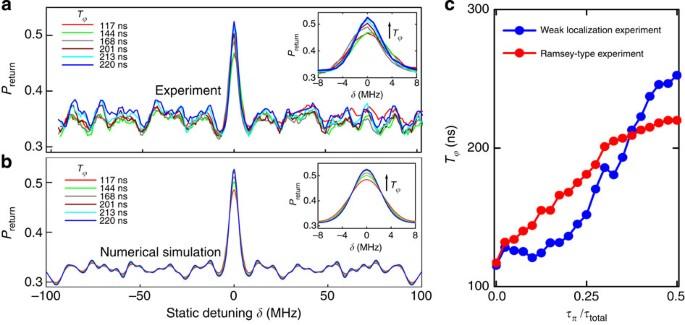Figure 2: Emulating the temperature dependence of weak localization. (a) Measured photon return probabilityPreturnas a function of the static detuningδ(simulating a magnetic field), for six different effective coherence times. ThePreturnpeak at zero detuning is analogous to the magnetoresistance peak associated with weak localization. Inset shows a magnified view ofPreturnnearδ=0, where we can observe the growth of thePreturnpeak. This emulates the growth of the magnetoresistance peak when lowering the temperature. (b) The photon return probabilityPreturnas a function ofδobtained through numerical calculations, at the same six different effective coherence timeas the experiment. (c) The effective coherence timeextracted from the experiments, in comparison withdirectly measured by Ramsey-type experiments, as a function ofτπ/τtotal. Figure 2: Emulating the temperature dependence of weak localization. ( a ) Measured photon return probability P return as a function of the static detuning δ (simulating a magnetic field), for six different effective coherence times . The P return peak at zero detuning is analogous to the magnetoresistance peak associated with weak localization. Inset shows a magnified view of P return near δ =0, where we can observe the growth of the P return peak. This emulates the growth of the magnetoresistance peak when lowering the temperature. ( b ) The photon return probability P return as a function of δ obtained through numerical calculations, at the same six different effective coherence time as the experiment. ( c ) The effective coherence time extracted from the experiments, in comparison with directly measured by Ramsey-type experiments, as a function of τ π / τ total . Full size image With the basic phenomena established, we focus on the small detuning region to investigate the role of quantum coherence, through variations in ( Fig. 2a inset). While the overall structure remains unchanged, the peak in P return grows as is increased; the peak rises from ~0.46 for to ~0.53 for , consistent with the temperature dependence of weak localization, where lower temperatures and thus longer phase coherence lengths increase the magnitude of the negative magnetoresistance peak [28] . As they are performed on a highly controlled quantum system, our experimental results can be understood within the Tavis–Cummings model (see Supplementary Note 1 ). As shown in Fig. 2b , we numerically evaluated P return versus δ , using the same six as in the experiment. In the calculations we have also included the energy dissipation time for each qubit, T 1 ~500 ns. Except for details in the aperiodic structures, the numerical results agree remarkably well with our experimental observations. Just as the phase coherence length L φ can be extracted from magnetoresistance measurements displaying weak localization, we can extract the effective coherence time from our measured P return ( δ ). We measured P return ( δ =0) for various τ π / τ total , and subsequently extracted from the height of the P return peak, based on the relationship (see Supplementary Note 1 ). The result is shown in Fig. 2c , compared with determined using conventional Ramsey-type measurements. As τ π / τ total increases from 0 to 0.5, increases as expected due to the cancellation of the qubit frequency drifts. We find reasonable agreement between the values of as measured with the two techniques, with deviations possibly caused by the finite number of ensembles in the emulation. In Supplementary Fig. 3 , we demonstrate we can also emulate the temperature dependence of weak antilocalization. Emulating disorder effects on weak localization The importance of the weak localization effect is not only because it reveals quantum coherence in transport, but also because it is a precursor to strong localization, also known as Anderson localization [29] . In the diffusive regime where weak localization manifests, the electron displacement at a given time has a Gaussian distribution whose width depends on the level of disorder. With an increasing disorder, the electron encounters more frequent scattering, resulting in a narrower distribution of its displacement. In the strong disorder limit, quantum interference completely halts carrier transmission, producing a disorder-driven metal-to-insulator transition. To measure the return probability P return as a function of disorder, we average 100 random detuning pulse sequences with different distributions of τ total , where τ total is randomly generated from a Gaussian distribution with width σ . Correlating the disorder with σ , we simulate weak localization at increasing disorder levels by reducing σ from 100 to 50 to 25 ns. In this way, we directly and separately tune the level of disorder, in contrast with the mesoscopic system where tuning the disorder level typically changes other parameters such as carrier density [30] , [31] , [32] . We note that adjusting σ by itself is only valid for emulating disorder in our special case, where only time-reversed symmetric pairs are considered in the emulation. For a more complete emulation where cross-interference is included, the value of τ R should also be reduced in proportion to τ total to account for more frequent scattering events. The experimentally measured P return versus δ for these three emulated disorder levels is shown in Fig. 3a . While the baseline value remains unchanged, the height of the zero-detuning peak grows as we reduce σ . This growth in the peak height with smaller σ agrees with the observation that an increased degree of disorder enhances localization in electron transport [30] , [31] , [32] . 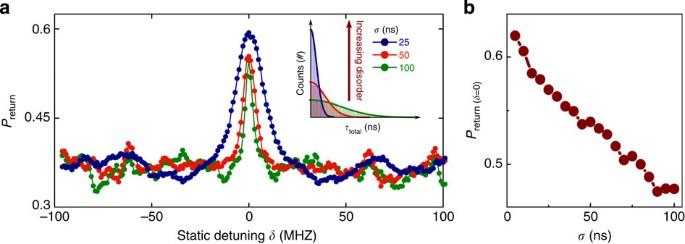Figure 3: Emulating the disorder dependence of weak localization. (a) Inset: Three distributions used forτtotalvalues, with standard deviationsσ=100, 50 and 20 ns. Main panel:Preturnas a function ofδfor the distributions shown in the inset. (b)Preturnat zero detuning as a function of the distribution width, showing the return probability increasing as the distribution is reduced. Figure 3: Emulating the disorder dependence of weak localization. ( a ) Inset: Three distributions used for τ total values, with standard deviations σ =100, 50 and 20 ns. Main panel: P return as a function of δ for the distributions shown in the inset. ( b ) P return at zero detuning as a function of the distribution width, showing the return probability increasing as the distribution is reduced. Full size image To find the signature of a disorder-driven metal–insulator transition, we focus on P return at δ =0 while continuously reducing σ . The results, using τ π / τ total =0.5 for maximum , are displayed in Fig. 3b . Reducing σ results in an increase of the photon return probability, with P return ( δ =0) increasing from 0.47 at σ =200 ns to 0.62 at σ =10 ns. However, there is no clear indication of an abrupt transition to a fully localized state, which would correspond to P return approaching unity. The metal–insulator transition is therefore not observed in our current experiment. Observing this transition likely requires further increasing the level of disorder by further increase of the ratio . Such studies are now possible using the recent 100-fold improvement in coherence time in the Xmon transmon qubit [33] , and are currently underway. Our experiment demonstrates that a few-element quantum circuit can be used to emulate the basics of weak localization. We demonstrate that we can achieve the required level of control to complete the emulation. These operations can in principle be extended to perform the emulation on a large-scale quantum circuit, which might shed light on more profound aspects of weak localization, such as its dependence on system dimensionality as well as to explore the effects of electron–electron interactions [34] . There are aperiodic structures at the baseline of P return that appear in both the experimental and numerical results. The shape of these structures is independent of , while the fluctuation amplitude increases with increasing . These resemble the universal conductance fluctuations associated with weak localization in mesoscopic systems [35] , [36] , [37] and are consistent with the previous experiment using a driven flux qubit [23] . Our experiment, however, does not include the cross-interference terms between trajectories that do not have time-reversed symmetry, so it is unclear if the fluctuation amplitudes here have a universal value independent of the experimental details. Emulation using a larger quantum circuit would be needed to clarify this issue. The quantum circuit used in this experiment uses the same circuit design as that used to implement Shor’s algorithm [24] . As shown in Fig. 1b , it is composed of four superconducting phase qubits, each connected to a memory resonator and all symmetrically coupled to a single central coupling resonator. The chip was fabricated using conventional multilayer lithography and reactive ion etching. The different metal Al layers were deposited using DC sputtering and the low-loss dielectric α -Si was deposited using plasma-enhanced chemical vapour deposition. The flux-biased phase qubit includes a 1pF parallel plate capacitor and a 700pH double-coiled inductor shunted with a Al/AlOx/Al Josephson junction. The phase qubit can be modelled as a nonlinear LC oscillator, whose nonlinearity arises from the Josephson junction. Adjusting the flux applied to the qubit loop, we can modulate the phase across the junction and consequently tune the qubit frequency. We are thus able to tune the qubit frequency over more than several hundred MHz without introducing any significant variation in the qubit phase coherence. This property is crucial for this implementation of the simulation protocol. How to cite this article: Chen, Y. et al. Emulating weak localization using a solid-state quantum circuit. Nat. Commun. 6:5184 doi: 10.1038/ncomms6184 (2014).